Ciliopathy-associated geneCc2d2apromotes assembly of subdistal appendages on the mother centriole during cilia biogenesis The primary cilium originates from the mother centriole and participates in critical functions during organogenesis. Defects in cilia biogenesis or function lead to pleiotropic phenotypes. Mutations in centrosome-cilia gene CC2D2A result in Meckel and Joubert syndromes. Here we generate a Cc2d2a −/− mouse that recapitulates features of Meckel syndrome including embryonic lethality and multiorgan defects. Cilia are absent in Cc2d2a −/− embryonic node and other somatic tissues; disruption of cilia-dependent Shh signalling appears to underlie exencephaly in mutant embryos. The Cc2d2a −/− mouse embryonic fibroblasts (MEFs) lack cilia, although mother centrioles and pericentriolar proteins are detected. Odf2, associated with subdistal appendages, is absent and ninein is reduced in mutant MEFs. In Cc2d2a −/− MEFs, subdistal appendages are lacking or abnormal by transmission electron microscopy. Consistent with this, CC2D2A localizes to subdistal appendages by immuno-EM in wild-type cells. We conclude that CC2D2A is essential for the assembly of subdistal appendages, which anchor cytoplasmic microtubules and prime the mother centriole for axoneme biogenesis. The primary cilium is a ubiquitous microtubule (MT)-based organelle, projecting from the cell surface to perform specialized sensory and signalling functions during organogenesis and cellular/tissue homeostasis [1] , [2] , [3] . In quiescent or post-mitotic cells, the migration of the centrosome towards the plasma membrane sets the stage for biogenesis of the primary cilium, which originates from the mother centriole (MC) acting as the basal body [4] . The two centrioles in the centrosome are ultrastructurally distinct; only the MC has distal and subdistal appendages (SDA) [5] and is involved in membrane tethering/docking, whereas the daughter centriole anchors cytoplasmic MT arrays [6] . The formation of the ciliary axoneme is initiated at the distal end of MC by the docking of a primary ciliary vesicle followed by coordinated trafficking of hundreds of proteins including signalling molecules and receptors via MT motors and intraflagellar transport complexes [7] , [8] . The efforts to define critical steps in cilia biogenesis have intensified lately because of the association of ciliary function with human diseases. Given the commonalities in cilia and centrosomes and their nearly universal presence, it is not surprising that aberrant cilia biogenesis and/or function can impact multiple tissues and cell types and manifest as pleiotropic syndromic disorders, collectively termed ciliopathies [9] , [10] , [11] , [12] . The ciliopathies encompass a spectrum of clinically distinguishable phenotypes that include retinal degeneration, cognitive impairment, neural tube defects, hydrocephalus, polycystic kidney, polydactyly, situs inversus and obesity. The clinical findings could include blindness (as in Leber congenital amaurosis) and/or cystic kidneys (as in nephronophthesis) as the primary manifestation. Alternately, the phenotypes can encompass multiple system defects as in Bardet–Biedl syndrome and Joubert syndrome (JBTS) or appear as a rare lethal malformation in Meckel syndrome (MKS). Strikingly, similar syndromic disorders can result from mutations in many different genes, and mutations in one gene can lead to distinct clinical manifestations. The observed phenotypic diversity in ciliopathies might also reflect a cumulative genetic load of variants/mutations and interactions among cilia-associated genes [12] , [13] , [14] . The search for homozygous genomic regions in 10 unrelated MKS fetuses led to the identification of the ciliopathy gene, CC2D2A [15] , which was independently discovered by homozygosity mapping of consanguineous families with JBTS [16] . Concurrently, a third group reported a homozygous splice site mutation in a large Pakistani family with mental retardation and retinitis pigmentosa [17] . Follow-up studies suggest that CC2D2A mutations in JBTS patients are less deleterious than those causing MKS [18] . CC2D2A encodes a coiled coil and C2 domain containing protein that is required for cilia formation and predicted to be involved in calcium-dependent membrane targeting [15] . The CC2D2A protein also includes a catalytically inactive version of the transglutaminase-like domain that may provide a peptide-binding interface for MTs [19] . CC2D2A is localized to the basal body and can physically interact with CEP290 (ref. 16) [16] , a cilia-centrosomal protein associated with numerous ciliopathies [20] . Interestingly, the multiprotein complex containing Tectonic1, associated with regulation of Hedgehog signalling, includes both CC2D2A and CEP290, and these proteins have been localized to the transition zone between the basal body and ciliary axoneme [21] . A fundamental requirement of CC2D2A in organogenesis is implied from embryonic lethality in human MKS [15] . The fibroblasts derived from a MKS embryo harbouring a CC2D2A mutation are unable to extend ciliary axoneme even though the basal body (that is, MC) is present, suggesting an essential role of CC2D2A in cilia biogenesis [15] . Nevertheless, a nonsense cc2d2a mutation identified in the sentinel zebrafish mutant did not reveal defects in motile cilia number or morphology, although some JBTS-like phenotypes (such as pronephric cysts) were detected [16] . To elucidate the function of CC2D2A in cilia biogenesis and produce a model of MKS, we generated a Cc2d2a -null allele in mice. The loss of Cc2d2a ( Cc2d2a −/− ) results in embryonic lethality with multiorgan defects related to cilia biogenesis. We show that CC2D2A localizes to the SDA in the MC and its loss prevents the assembly of SDA and anchoring of MTs. Our studies further delineate the fundamental sequence of cilia biogenesis from the MC and uncover ciliary ultrastructural defects associated with the loss of CC2D2A function in MKS. The loss of Cc2d2a in mouse leads to embryonic lethality Three protein-coding transcript variants are produced from the Cc2d2a gene. To eliminate all transcripts, we replaced Cc2d2a exons 6 to 8, shared by all variants, with a targeting vector containing a β-gal reporter and a neomycin selection cassette ( Fig. 1a ) through standard homologous recombination in ES cells. Southern blotting of genomic DNA from ES clones using an exon 5–6 probe ( Fig. 1a ) showed 12.7 and 9.9 kb Eco RI fragments for the wild-type and Cc2d2a −/− alleles, respectively ( Fig. 1b , Supplementary Fig. 1 ). We confirmed that the embryos homozygous for the targeted allele (indicated as −/− or Cc2d2a −/− ) lacked the Cc2d2a transcript ( Fig. 1c ). Finally, we demonstrated by immunoblot analysis that Cc2d2a −/− embryos lacked the CC2D2A protein ( Fig. 1d , Supplementary Fig. 2 ). 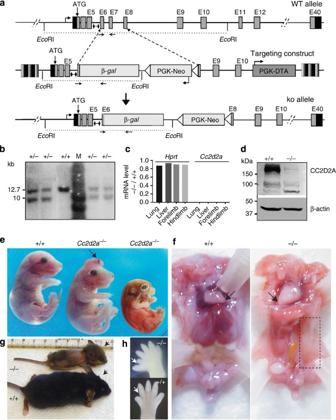Figure 1: The loss ofCc2d2aleads to embryonic lethality with pleiotropic defects in organogenesis. (a) The design for generatingCc2d2aknockout (ko) allele in mouse. The wild-typeCc2d2alocus at mouse chromosome 5 (top), the targeting vector (middle) and the ko allele (bottom) are shown. Small lines with diamond caps indicate the DNA fragment used as a probe for Southern blot analysis. Mice were genotyped using the forward and reverse primers indicated by arrows. (b) Validation ofCc2d2ako allele in ES cells by Southern blot analysis after digestion withEcoRI, as shown ina. Successful recombination with the targeting vector would yield both wild-type (12.7 kb) and targeted (9.9 kb) fragments. M, DNA ladder; +, wild type allele; −, ko allele. (c) Reverse transcriptase PCR analysis ofCc2d2atranscripts. The ratio ofHprt(control) orCc2d2atranscripts in −/− versus +/+ tissues of newborn (P0) mouse is shown. Cc2d2atranscripts were undetectable in the ko embryos. (d) Immunoblot analysis with anti-CC2D2A antibody on protein extract from the wild-type andCc2d2ako embryos aged E14. A 187 kDa CC2D2A protein was detected in the wild type (+/+), whereas in the −/− embryos CC2D2A was undetectable. β-Actin was used as a loading control. (e) Gross phenotype of E16Cc2d2a−/−embryos compared with wild type (+/+) littermates. Mutant embryos display a range of developmental defects, including exencephaly or open rostral neural tube (arrow; middle), small size (right) and microphthalmia (dotted oval). (f) Visceral phenotype ofCc2d2a−/−embryos. The −/− embryos display dextrocardia (arrow) and this one lacks kidney, spleen on the left side, in addition to large part of intestine (dotted rectangle). (g) The phenotype of a single rare −/− survivor at P27, along with its littermate control. The −/− (top) animal has a domed head representing profound hydrocephalus compared with its +/+ littermate (lower). See alsoSupplementary Fig. 3. (h) Hind limbs from wild-type and −/− embryos. Note the pre-axial polydactyly on the hind limb of −/− embryo (arrow). Figure 1: The loss of Cc2d2a leads to embryonic lethality with pleiotropic defects in organogenesis. ( a ) The design for generating Cc2d2a knockout (ko) allele in mouse. The wild-type Cc2d2a locus at mouse chromosome 5 (top), the targeting vector (middle) and the ko allele (bottom) are shown. Small lines with diamond caps indicate the DNA fragment used as a probe for Southern blot analysis. Mice were genotyped using the forward and reverse primers indicated by arrows. ( b ) Validation of Cc2d2a ko allele in ES cells by Southern blot analysis after digestion with Eco RI, as shown in a . Successful recombination with the targeting vector would yield both wild-type (12.7 kb) and targeted (9.9 kb) fragments. M, DNA ladder; +, wild type allele; −, ko allele. ( c ) Reverse transcriptase PCR analysis of Cc2d2a transcripts. The ratio of Hprt (control) or Cc2d2a transcripts in −/− versus +/+ tissues of newborn (P0) mouse is shown . Cc2d2a transcripts were undetectable in the ko embryos. ( d ) Immunoblot analysis with anti-CC2D2A antibody on protein extract from the wild-type and Cc2d2a ko embryos aged E14. A 187 kDa CC2D2A protein was detected in the wild type (+/+), whereas in the −/− embryos CC2D2A was undetectable. β-Actin was used as a loading control. ( e ) Gross phenotype of E16 Cc2d2a −/− embryos compared with wild type (+/+) littermates. Mutant embryos display a range of developmental defects, including exencephaly or open rostral neural tube (arrow; middle), small size (right) and microphthalmia (dotted oval). ( f ) Visceral phenotype of Cc2d2a −/− embryos. The −/− embryos display dextrocardia (arrow) and this one lacks kidney, spleen on the left side, in addition to large part of intestine (dotted rectangle). ( g ) The phenotype of a single rare −/− survivor at P27, along with its littermate control. The −/− (top) animal has a domed head representing profound hydrocephalus compared with its +/+ littermate (lower). See also Supplementary Fig. 3 . ( h ) Hind limbs from wild-type and −/− embryos. Note the pre-axial polydactyly on the hind limb of −/− embryo (arrow). Full size image The analysis of F2 litters produced by crossing heterozygous Cc2d2a +/− mice identified live pups with only Cc2d2a +/+ and Cc2d2a +/− genotypes, suggesting lethality of Cc2d2a −/− homozygous-null embryos. We then assessed at what age Cc2d2a −/− embryos are lost. We were able to identify Cc2d2a −/− embryos at close to predicted ratios (25%) on embryonic day (E) 14 and E16. However, the ratio of Cc2d2a −/− embryos declined sharply at E18 (to 4%), and null mutants rarely survived beyond that age ( Table 1 ). At E16–18, Cc2d2a −/− embryos displayed pleiotropic phenotypes resembling MKS, with many showing severe degeneration and resorption during early embryogenesis ( Fig. 1e ). In addition to haemorrhage, open neural tube, microphthalmia, and anophthalmia, Cc2d2a −/− embryos often revealed situs inversus and dextrocardia, and on occasion, lacked abdominal organs ( Fig. 1f , boxed area). Polydactyly was observed frequently in Cc2d2a −/− embryos ( Fig. 1h , arrows). Thus, Cc2d2a is broadly required for organogenesis in mice. Among hundreds of Cc2d2a −/− mutants generated in our laboratory, only one mouse survived for 27 days and showed gross underdevelopment with marked lethargy, loss of hair on its dorsal surface, hydrocephalus ( Fig. 1g , compare arrows), and retinal dystrophy ( Supplementary Fig. 3 ). Table 1 Genotypes obtained from heterozygous ( +/− ) interbreeding. Full size table Cc2d2a −/− embryos have defects in motile and sensory cilia The situs inversus phenotype suggested defects in the embryonic node and establishment of left–right asymmetry. Scanning electron microscopy of the E8 Cc2d2a −/− embryos revealed flattening of the node with only a few cilia-like structures ( Fig. 2a–c ). Immunostaining of the embryonic node using anti-acetylated α-tubulin antibody validated these findings ( Fig. 2d ). The analysis of other ciliated tissues also showed profound defects in cilia biogenesis. The kinocilia in the cochlea were frequently absent or abnormal (green signal in Fig. 2e , right) and stereociliary bundles deformed (red signal in Fig. 2e , right) in Cc2d2a −/− embryos. The cilia were also absent or abnormal in Cc2d2a −/− embryonic liver (green signal in Fig. 2f , right). Perinatal kidney tubules and tracheal epithelium revealed few cilia in Cc2d2a −/− embryos (green signal in Fig. 2g,h , right panels). By comparison, kidney tubules in wild-type embryos had prominent, primary cilia projecting into the lumen ( Fig. 2g , left), and tracheal epithelia presented tufts of motile cilia ( Fig. 2h , left). 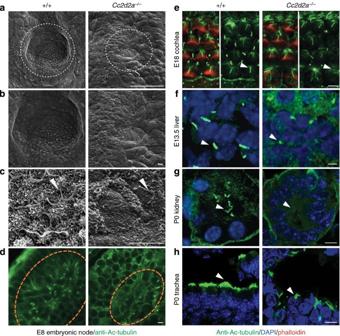Figure 2: Motile and sensory cilia biogenesis is defective inCc2d2a−/−embryos. (a–c) Scanning electron micrographs of E8 embryonic node in increasing order of magnification. The wild-type node comprises ciliated cells, whereas the −/− embryo had only rare cilia (arrowheads inc). (d) Immunostaining for cilia markers (anti-α-acetylated tubulin, green) on E8 embryonic node (within the dashed circled area). The wild-type embryo (left panel) had many cilia compared with the −/− embryo (right panel) that had almost none. (e) E18 cochlea showing kinocilia (anti-α-acetylated tubulin, green) and stereocilia (phalloidin, red) in wild-type (+/+) andCc2d2a−/−embryos. In the wild type, kinocilia were evenly spaced and aligned, whereas those in the −/− were missing or misoriented (arrowhead). (f) E13.5 liver from wild-type (+/+) andCc2d2a−/−embryos showing cilia staining (anti-α-acetylated tubulin, green). Cilia were underdeveloped in −/− liver (arrowheads). (g) Kidney tubule and (h) trachea from P0 wild-type (+/+) andCc2d2a−/−mice showing cilia staining (anti-α-acetylated tubulin, green). The wild-type kidney had many long luminal cilia that are not detected in the −/− mice (arrowheads). Similarly, the −/− trachea had no cilia (arrowheads) compared with tufts of multiple motile cilia on each epithelial cell in the wild type. The scale bars in all panels are 5 μm except in ‘a’, which is 50 μm. Ind–h, anti-α-acetylated tubulin is green and nuclear DAPI counterstain is blue. Figure 2: Motile and sensory cilia biogenesis is defective in Cc2d2a −/− embryos. ( a – c ) Scanning electron micrographs of E8 embryonic node in increasing order of magnification. The wild-type node comprises ciliated cells, whereas the −/− embryo had only rare cilia (arrowheads in c ). ( d ) Immunostaining for cilia markers (anti-α-acetylated tubulin, green) on E8 embryonic node (within the dashed circled area). The wild-type embryo (left panel) had many cilia compared with the −/− embryo (right panel) that had almost none. ( e ) E18 cochlea showing kinocilia (anti-α-acetylated tubulin, green) and stereocilia (phalloidin, red) in wild-type (+/+) and Cc2d2a −/− embryos. In the wild type, kinocilia were evenly spaced and aligned, whereas those in the −/− were missing or misoriented (arrowhead). ( f ) E13.5 liver from wild-type (+/+) and Cc2d2a −/− embryos showing cilia staining (anti-α-acetylated tubulin, green). Cilia were underdeveloped in −/− liver (arrowheads). ( g ) Kidney tubule and ( h ) trachea from P0 wild-type (+/+) and Cc2d2a −/− mice showing cilia staining (anti-α-acetylated tubulin, green). The wild-type kidney had many long luminal cilia that are not detected in the −/− mice (arrowheads). Similarly, the −/− trachea had no cilia (arrowheads) compared with tufts of multiple motile cilia on each epithelial cell in the wild type. The scale bars in all panels are 5 μm except in ‘ a ’, which is 50 μm. In d – h , anti-α-acetylated tubulin is green and nuclear DAPI counterstain is blue. Full size image Shh signalling is perturbed in Cc2d2a −/− embryos As Cc2d2a −/− embryos often exhibited exencephaly (see Fig. 1e ), we hypothesized that the open neural tube phenotype is due to abnormal cilia biogenesis and perturbed Shh signalling [22] , [23] , [24] . Our analysis of E 12 embryos revealed the presence of cilia in the neural tube in the wild type ( Fig. 3a , upper middle panel) but not in the Cc2d2a −/− mutants ( Fig. 3a , lower middle panel). We noted the presence of basal bodies in the neural tube of both genotypes ( Fig. 3a , left panels). 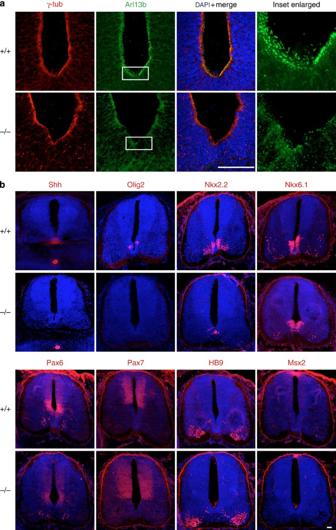Figure 3: Cilia-mediated Shh signalling is perturbed in the developing neural tube ofCc2d2a−/−embryos. (a) Immunostaining for anti-γ tubulin (marker of basal bodies; red) and anti-Arl13b (highlighting cilia; green) in embryonic (E12) neural tube. In wild-type embryo (+/+) neural tube showed presence of both basal bodies (red) and cilia (green). In ko embryo (−/−), the cilia are missing and the basal bodies are mislocalized. The inset region is enlarged and shown at the right. (b) Immunostaining for indicated markers (red) in embryonic E12 neural tube. In the wild type (+/+), the Shh signal was clearly seen in the ventral floor plate and notochord whereas in the ko (−/−) the Shh signal was absent in the floor plate. Olig2 and Nkx2.2 were both evident in ventral domains near the floor plate in the wild type, but in the mutant Olig2 was absent and Nkx2.2 was seen ectopically at the floor plate. Compared with the wild type, Nkx6.1 signal was shifted ventrally, and Pax6 domain also showed a slight expansion ventrally. Pax7, HB9 and the roof plate maker Msx2 did not show any apparent difference in signal intensity and pattern in the wild-type and the ko embryos. The nuclear staining is done with DAPI (blue). The images are taken in rostrocaudal axis approximately in the hind limb level. Scale bars, 50 μm. Figure 3: Cilia-mediated Shh signalling is perturbed in the developing neural tube of Cc2d2a −/− embryos. ( a ) Immunostaining for anti-γ tubulin (marker of basal bodies; red) and anti-Arl13b (highlighting cilia; green) in embryonic (E12) neural tube. In wild-type embryo (+/+) neural tube showed presence of both basal bodies (red) and cilia (green). In ko embryo (−/−), the cilia are missing and the basal bodies are mislocalized. The inset region is enlarged and shown at the right. ( b ) Immunostaining for indicated markers (red) in embryonic E12 neural tube. In the wild type (+/+), the Shh signal was clearly seen in the ventral floor plate and notochord whereas in the ko (−/−) the Shh signal was absent in the floor plate. Olig2 and Nkx2.2 were both evident in ventral domains near the floor plate in the wild type, but in the mutant Olig2 was absent and Nkx2.2 was seen ectopically at the floor plate. Compared with the wild type, Nkx6.1 signal was shifted ventrally, and Pax6 domain also showed a slight expansion ventrally. Pax7, HB9 and the roof plate maker Msx2 did not show any apparent difference in signal intensity and pattern in the wild-type and the ko embryos. The nuclear staining is done with DAPI (blue). The images are taken in rostrocaudal axis approximately in the hind limb level. Scale bars, 50 μm. Full size image We then investigated a potential defect in the patterning of neural tube domain markers due to lack of cilia-mediated Shh signalling. In wild-type embryos, Shh signal localizes to the floor plate of neural tube and at the notochord ( Fig. 3b ). In contrast, Cc2d2a −/− embryos lack Shh signal at the floor plate ( Fig. 3b ). In contrast to the wild-type embryos showing Nkx2.2 and Nkx6.1 expression ( Fig. 3b ) at the ventral neural tube, Nkx2.2 signal was found at the floor plate in the Cc2d2a −/− embryos and Nkx6.1 expressing domain shifted towards the ventral midline ( Fig. 3b ). Furthermore, the Pax6 domain also expanded ventrally. These data indicate the loss of floor plate cell fate and a reduction in V3 progenitors, which require high levels of Shh for induction. Olig2 signal, marking progenitors of the oligodendrocyte lineage that also depend on Shh signalling for induction, was absent in the Cc2d2a −/− embryos ( Fig. 3b ). We note that Pax7, HB9 and Msx2 showed no discernable difference in Cc2d2a −/− embryos compared with the wild type ( Fig. 3b ). Thus, the neural tube patterning defect of Cc2d2a −/− embryos mostly affects ventral cell fates, consistent with a perturbation of Shh signalling. The neural tube patterning defect in this mutant is similar to that of the Mks1 mutant [25] . Cc2d2a −/− fibroblasts have basal body but not ciliary axoneme To delineate the underlying defect in cilia biogenesis, we isolated and cultured mouse embryonic fibroblasts (MEFs) from Cc2d2a −/− mutants. Unlike MEFs from wild-type littermates ( Fig. 4a , upper panel), Cc2d2a −/− MEFs did not grow cilia on serum starvation ( Fig. 4a , lower panel). We, however, noted that ~\n10% of Cc2d2a −/− MEFs escaped this phenotype. Both Cc2d2a −/− and wild-type MEFs showed similar MC staining with γ-tubulin, yet Arl13b labelling was compromised in Cc2d2a −/− MEFs ( Fig. 4a ). In addition, MT staining with acetylated α-tubulin showed presence of axoneme in the wild type but not in Cc2d2a −/− MEFs; nonetheless, cytoplasmic MTs were visible in Cc2d2a −/− MEFs ( Fig. 4c,d ). These data suggest that ciliary axoneme biogenesis was not initiated from the MC in the absence of Cc2d2a . The mouse Cc2d2a transgene could rescue the axoneme assembly defect in Cc2d2a −/− MEFs ( Fig. 4b ; note that the non-transfected cells in the same field do not have cilia), demonstrating a direct role of CC2D2A in the genesis of cilia from the MC. 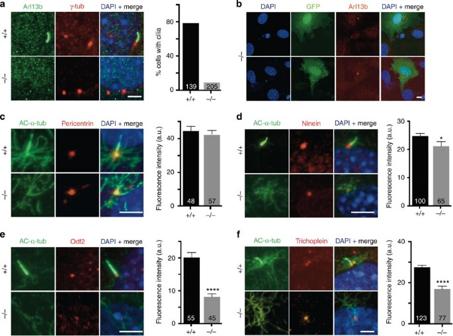Figure 4: Lack of cilia and defects in MC ofCc2d2a−/−MEFs can be rescued byCc2d2atransgene. (a)Cc2d2a−/−MEFs have MC but no cilia. Anti-Arl13b is used to highlight cilia. MC (basal body) is stained with γ-tubulin antibody. (b)Cc2d2atransgene rescues cilia biogenesis inCc2d2a−/−MEFs. Anti-Arl13b staining is shown in red circle. GFP (green) represents the transfected cells. Non-transfected cells in the same field do not have any cilia. Nuclei are stained with DAPI (blue). Inc,d, cilia are marked by acetylated α- tubulin (green). (c) Pericentrin (a proximal end marker of MC) staining (in red) is unaltered inCc2d2a−/−MEFs. See alsoSupplementary Fig. 4. (d) Immunostaining of ninein that marks both SDA and the MC proximal end is significantly reduced inCc2d2a−/−MEFs. (e) Anti-Odf2 immunostaining, which is detected at SDA in wild type, is barely visible inCc2d2a−/−MEFs. (f) Trichoplein immunostaining is reduced inCc2d2a−/−MEFs. Scale bars, 5 μm. Antibody is indicated above each panel. In merged images, blue nuclear stain is DAPI. The number of cells used for quantification is indicated in all graphs. The graph inacompares percentage of cells with cilia (yaxis) between wild-type (+/+) andCc2d2a−/−genotypes (xaxis). The graphs in remaining panels compare the level of antibody-generated fluorescence (red signal in each panel) between the two genotypes, wherexandyaxes are genotypes and corrected fluorescence intensity (arbitrary units, (a.u.)), respectively. Bars indicate s.e.m. The sample size (n) is indicated on the bar diagram, and the experiment was repeated three times.P-value was derived from unpaired two-tailedt-test. Statistical significance is marked with asterisks (* and **** indicateP≤0.05 and 0.0001, respectively). Figure 4: Lack of cilia and defects in MC of Cc2d2a −/− MEFs can be rescued by Cc2d2a transgene. ( a ) Cc2d2a −/− MEFs have MC but no cilia. Anti-Arl13b is used to highlight cilia. MC (basal body) is stained with γ-tubulin antibody. ( b ) Cc2d2a transgene rescues cilia biogenesis in Cc2d2a −/− MEFs. Anti-Arl13b staining is shown in red circle. GFP (green) represents the transfected cells. Non-transfected cells in the same field do not have any cilia. Nuclei are stained with DAPI (blue). In c , d , cilia are marked by acetylated α- tubulin (green). ( c ) Pericentrin (a proximal end marker of MC) staining (in red) is unaltered in Cc2d2a −/− MEFs. See also Supplementary Fig. 4 . ( d ) Immunostaining of ninein that marks both SDA and the MC proximal end is significantly reduced in Cc2d2a −/− MEFs. ( e ) Anti-Odf2 immunostaining, which is detected at SDA in wild type, is barely visible in Cc2d2a −/− MEFs. ( f ) Trichoplein immunostaining is reduced in Cc2d2a −/− MEFs. Scale bars, 5 μm. Antibody is indicated above each panel. In merged images, blue nuclear stain is DAPI. The number of cells used for quantification is indicated in all graphs. The graph in a compares percentage of cells with cilia ( y axis) between wild-type (+/+) and Cc2d2a −/− genotypes ( x axis). The graphs in remaining panels compare the level of antibody-generated fluorescence (red signal in each panel) between the two genotypes, where x and y axes are genotypes and corrected fluorescence intensity (arbitrary units, (a.u. )), respectively. Bars indicate s.e.m. The sample size (n) is indicated on the bar diagram, and the experiment was repeated three times. P -value was derived from unpaired two-tailed t -test. Statistical significance is marked with asterisks (* and **** indicate P ≤0.05 and 0.0001, respectively). Full size image The existence of a MC but lack of axoneme suggested that Cc2d2a is needed in early ciliogenic processes. After polarity-guided centriolar migration, the MC docks to the membrane with distal appendages, whereas the anchoring of MT arrays requires SDA [6] . Even though MT nucleation starts with aster formation at both centrioles, only the MC is able to sustain a stable MT array, a process requiring ninein [26] , [27] . Immunolabelling with anti-ninein antibody revealed a significant reduction of ninein signal at the MC in Cc2d2a −/− MEFs ( Fig. 4d ). It should be noted that ninein is present predominantly at the distal end of the MC, on SDA, while it is also detectable at the proximal ends of both centrioles. Our results thus indicate a basic structural defect in the MC. Distal end components are abnormal in MC of Cc2d2a −/− MEFs Immunolabelling of wild-type and Cc2d2a −/− MEFs using rootletin and pericentrin antibodies revealed no significant differences ( Fig. 4c and Supplementary Fig. 4a ), implying structural integrity of pre-proximal and proximal ends of the two centrioles. Absence of the ciliary axoneme and reduced ninein staining prompted us to examine Odf2, an established marker of SDA [28] , which is needed for cilia biogenesis [29] . The anti-Odf2 signal at the MC was dramatically reduced in Cc2d2a −/− MEFs compared with the wild type ( Fig. 4e ). We then performed immunolabelling against trichoplein, which controls MT anchoring at the MC by binding to Odf2 and ninein [30] . Interestingly, trichoplein signal was also significantly reduced at the MC in Cc2d2a −/− MEFs ( Fig. 4f ). Our results suggest that recruitment of Odf2 and trichoplein to the SDA is compromised when CC2D2A is not present, and that CC2D2A is needed for SDA assembly. CC2D2A is required to form SDA The loss of cc2d2a in zebrafish photoreceptors resulted in mislocalization of Rab8 (ref. 31) [31] , which interacts with Odf2 and is needed for cilia biogenesis [32] . In Cc2d2a −/− MEFs, Rab8 staining is significantly reduced compared with the wild type ( Fig. 5a ). Furthermore, transfection of Rab8a-mCherry in wild-type MEFs showed sharp localization at the base of the cilium, whereas the signal was diffuse and cytoplasmic in Cc2d2a −/− MEFs ( Fig. 5b ). Notably, immunoblotting demonstrated similar levels of Rab8a protein in the wild-type and Cc2d2a −/− MEFs ( Supplementary Fig. 5 ). These results thus indicate defective vesicle docking or membrane tethering at the MC in the absence of CC2D2A. 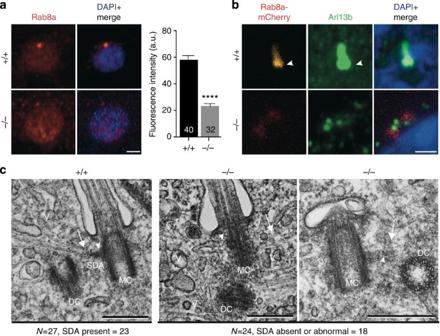Figure 5: Accumulation of transport vesicles and lack of or abnormal SDA inCc2d2a−/−MEFs. (a) Immunostaining of Rab8a (red) that marks transport vesicles in wild-type andCc2d2a−/−MEFs. Rab8a localization is diffuse in cytoplasm inCc2d2a−/−MEFs compared with the wild type. Thexandyaxes are genotypes and corrected fluorescence intensity (arbitrary units, (a.u.)), respectively. Bars indicate s.e.m. Signal intensity quantification shows a highly significant difference (P-value was derived from unpaired two tailedt-test; **** indicatesP-value ≤0.0001). The sample size (n) is indicated on the bar diagram, and the experiment was repeated three times. (b) Immunostaining for anti-Arl13b (green) and Rab8a-mCherry (red) transfected in wild-type andCc2d2a−/−MEFs. Rab8a-mCherry signal is sharp at the base of the cilium (arrowhead) in wild-type cells but diffuse in −/− MEFs. Nuclei are stained with DAPI (blue). (c) Transmission electron micrographs of cilia from wild-type andCc2d2a−/−MEFs. In wild type, the MC has well-defined SDA (arrow head), to which MTs (arrow) are anchored for trafficking of vesicles (V). InCc2d2a−/−MEFs, the SDA is not visible at a comparable location (middle panel, arrowhead) or an abnormal SDA with compromised transition zone (right panel, arrowhead) and the MTs (arrow) are not anchored. The vesicles accumulate in the cytoplasm around the MC. The total number (N) of MEFs analysed for the presence of SDA or abnormal SDA is indicated. MC and daughter centriole (DC) are mother and daughter centriole, respectively. Scale bars inaandbare 5 μm and incis 500 nm. Figure 5: Accumulation of transport vesicles and lack of or abnormal SDA in Cc2d2a −/− MEFs. ( a ) Immunostaining of Rab8a (red) that marks transport vesicles in wild-type and Cc2d2a −/− MEFs. Rab8a localization is diffuse in cytoplasm in Cc2d2a −/− MEFs compared with the wild type. The x and y axes are genotypes and corrected fluorescence intensity (arbitrary units, (a.u. )), respectively. Bars indicate s.e.m. Signal intensity quantification shows a highly significant difference ( P -value was derived from unpaired two tailed t -test; **** indicates P -value ≤0.0001). The sample size ( n ) is indicated on the bar diagram, and the experiment was repeated three times. ( b ) Immunostaining for anti-Arl13b (green) and Rab8a-mCherry (red) transfected in wild-type and Cc2d2a −/− MEFs. Rab8a-mCherry signal is sharp at the base of the cilium (arrowhead) in wild-type cells but diffuse in −/− MEFs. Nuclei are stained with DAPI (blue). ( c ) Transmission electron micrographs of cilia from wild-type and Cc2d2a −/− MEFs. In wild type, the MC has well-defined SDA (arrow head), to which MTs (arrow) are anchored for trafficking of vesicles (V). In Cc2d2a −/− MEFs, the SDA is not visible at a comparable location (middle panel, arrowhead) or an abnormal SDA with compromised transition zone (right panel, arrowhead) and the MTs (arrow) are not anchored. The vesicles accumulate in the cytoplasm around the MC. The total number ( N ) of MEFs analysed for the presence of SDA or abnormal SDA is indicated. MC and daughter centriole (DC) are mother and daughter centriole, respectively. Scale bars in a and b are 5 μm and in c is 500 nm. Full size image To further investigate cellular ultrastructure at and near the MC, we took advantage of transmission electron microscopy (TEM). In wild-type MEFs, normal ciliary structures were evident with MTs anchored at SDA and oriented in a regular array from the cytoplasm towards the basal body ( Fig. 5c ; left, arrow). However, in Cc2d2a −/− MEFs, the MC lacked or had abnormal SDA, had disorganized MTs and showed accumulation of vesicle-like structures nearby ( Fig. 5c , middle panel). Notably, in a fraction of Cc2d2a −/− MEFs, the MC docked to ciliary vesicles but apparently no transition zone developed ( Fig. 5c , right panel). This finding was not obtained in the wild-type MEFs. We therefore conclude that CC2D2A is needed for the assembly of SDA at MC, for stable MT anchoring and docking of transport vesicles, and for further elaboration of the transition zone. MT regrowth assays using α- and γ-tubulin [33] were then performed to evaluate whether MT anchoring at the MC requires CC2D2A. In wild-type and Cc2d2a −/− MEFs, MT regrowth did not initiate immediately after removing nocodazole ( Fig. 6 , 0 min). At 5 min, the MT started reappearing at the MC in the wild type, but not seen in Cc2d2a −/− MEFs. At 30 min of recovery from nocodazole MT aster anchoring at the MC was visible in wild-type cells ( Fig. 6 , 30 min). At 30 min, although MTs were visible in Cc2d2a −/− MEFs, these did not form an aster and anchor at the basal body. These data demonstrate a critical role of CC2D2A in MT anchoring at the basal body. 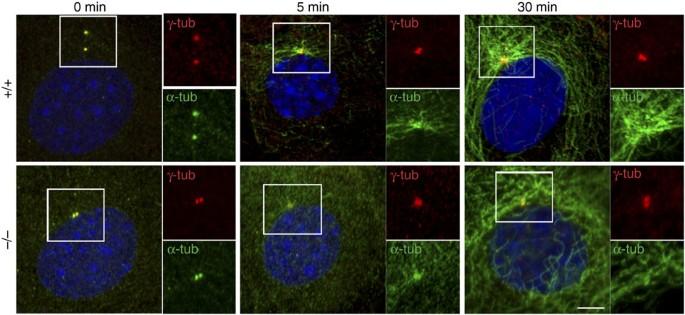Figure 6: CC2D2A is required for MT anchoring at the basal body. The MT array (α-tubulin, green) formation at the basal body (γ-tubulin, red) is not visible at 0 min in the wild-type (+/+) and the ko cells (−/−). At 5 min, the MT array is apparent at the basal body in the wild-type cells but not in the ko cells. At 30 min, a profuse array of MT forming an aster is observed at the basal body in the wild type but not in the ko cells even though cytoplasmic MTs are detected. The area in the inset is shown at the higher magnification on the right side of each image. Scale bar, 5 μm. Figure 6: CC2D2A is required for MT anchoring at the basal body. The MT array (α-tubulin, green) formation at the basal body (γ-tubulin, red) is not visible at 0 min in the wild-type (+/+) and the ko cells (−/−). At 5 min, the MT array is apparent at the basal body in the wild-type cells but not in the ko cells. At 30 min, a profuse array of MT forming an aster is observed at the basal body in the wild type but not in the ko cells even though cytoplasmic MTs are detected. The area in the inset is shown at the higher magnification on the right side of each image. Scale bar, 5 μm. Full size image CC2D2A localizes to SDA Immunolabelling in ciliated IMCD3 cells revealed the localization of CC2D2A protein to the MC. The CC2D2A staining partially overlapped with RPGR, a cilia transition zone marker [34] , and anti-GT335 ( Fig. 7a,b ), which labels polyglutamylated tubulin and marks both the basal body and the proximal axoneme [35] , [36] . Interestingly, CC2D2A immunostaining appeared similar to that of centriolin [35] and Odf2 (ref. 28) [28] . To further refine the localization of CC2D2A, we took advantage of immuno-EM. Immunogold labelling for CC2D2A was clearly visible on the SDA both in IMCD3 cells and in monkey retina ( Fig. 7c,d ). Our data are concordant with preceding MEF studies and strengthen the proposition of a role for CC2D2A in SDA assembly. 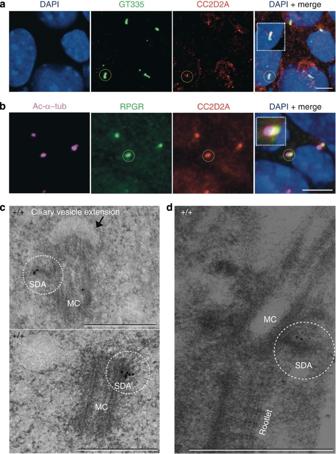Figure 7: CC2D2A localizes to SDA where ciliary transition zone begins. (a) Immunostaining for anti-GT335 (green) and anti-CC2D2A (red) in IMCD3 cells that were induced to generate cilia. Anti-GT335 signal marks the MC and the proximal part of the axoneme, whereas anti-CC2D2A staining is restricted to the MC (third panel, circled). Inset shows magnified view of the circled cilium. (b) Immunostaining for anti-α-acetylated tubulin (magenta), anti-RPGR (green) and anti-CC2D2A (red) in IMCD3 cells. RPGR is a cilia transition zone marker. The CC2D2A immunostaining partially overlaps with anti-RPGR signal (circled, enlarged in inset) at the base of axoneme marked by anti-α-acetylated tubulin. Nuclei are stained with DAPI (blue) inaandb. (c) Immuno-EM of MCs labelled with anti-CC2D2A from ciliated IMCD3 cells. Gold particles (10 nm) are localized to SDA on MC in both micrographs. The upper micrograph shows a ciliary vesicle of an extending cilium axoneme (arrow). (d) Immuno-EM of a monkey retina, using CC2D2A antibody inc. The gold particles align on the SDA. MC is supported by a rootlet. Scale bars inaandbare 5 μm, andcanddare 500 nm. Figure 7: CC2D2A localizes to SDA where ciliary transition zone begins. ( a ) Immunostaining for anti-GT335 (green) and anti-CC2D2A (red) in IMCD3 cells that were induced to generate cilia. Anti-GT335 signal marks the MC and the proximal part of the axoneme, whereas anti-CC2D2A staining is restricted to the MC (third panel, circled). Inset shows magnified view of the circled cilium. ( b ) Immunostaining for anti-α-acetylated tubulin (magenta), anti-RPGR (green) and anti-CC2D2A (red) in IMCD3 cells. RPGR is a cilia transition zone marker. The CC2D2A immunostaining partially overlaps with anti-RPGR signal (circled, enlarged in inset) at the base of axoneme marked by anti-α-acetylated tubulin. Nuclei are stained with DAPI (blue) in a and b . ( c ) Immuno-EM of MCs labelled with anti-CC2D2A from ciliated IMCD3 cells. Gold particles (10 nm) are localized to SDA on MC in both micrographs. The upper micrograph shows a ciliary vesicle of an extending cilium axoneme (arrow). ( d ) Immuno-EM of a monkey retina, using CC2D2A antibody in c . The gold particles align on the SDA. MC is supported by a rootlet. Scale bars in a and b are 5 μm, and c and d are 500 nm. Full size image No cell cycle defect in Cc2d2a −/− MEFs We detected similar anti-GT335 immunostaining in wild-type and Cc2d2a −/− MEFs ( Supplementary Fig. 4b , lower panels), consistent with the hypothesis that CC2D2A includes a catalytically inactive transglutaminase-like domain [19] . To test whether CC2D2A might be required for sensing Ca 2+ level changes during cell cycle [37] , we analysed the cell cycle profile in MEFs. No significant difference was identified between the wild-type and Cc2d2a −/− MEFs ( Supplementary Fig. 6 ). Embryonic lethality observed in MKS represents the most severe of all phenotypes in ciliopathies. CC2D2A is one of the 10 centrosome-cilia genes associated with MKS. Mutations in CC2D2A also cause JBTS, another relatively severe disease with a plethora of clinical findings. Previous studies implicate a fundamental role of CC2D2A in cilia biogenesis that when interrupted would lead to MKS or JBTS. However, the precise disease mechanism and CC2D2A function have been elusive. Here, we demonstrate that CC2D2A is required for the assembly of SDA that are critical for anchoring of MTs, vesicle docking and initiation of ciliary axoneme. Loss of CC2D2A, as in the Cc2d2a −/− embryos reported here, appears to prevent cilia-mediated functions of motile or sensory cilia, thereby leading to defects in organogenesis in MKS. We suggest that the less severe JBTS ciliopathy phenotype likely results from residual function of certain mutant CC2D2A alleles or from partial compensation by a modifier gene [14] , [38] , [39] . The Cc2d2a −/− mouse model recapitulates the phenotype reported in human MKS fetuses that inherit a nonsense mutation in CC2D2A [15] . The lethality observed in cc2d2a -null mutants of zebrafish [40] reflects the evolutionary conservation of Cc2d2a function in cilia biogenesis. Interestingly, although a Cc2d2a gene-trap mouse exhibits embryonic lethality, the MEFs derived from this mutant could extend a ciliary axoneme [21] , suggesting that the gene-trap allele may not be a complete null. Different mouse mutants therefore offer an opportunity to better elucidate underlying cilia biogenesis defects and pathologies in distinct syndromes caused by mutations in CC2D2A . We note that the situs inversus phenotype in Cc2d2a −/− embryos can be explained by the lack of nodal cilia, as in IFT-defective Kif3b mice [41] . However, the cilia defects are remarkably different in Cc2d2a −/− mutants compared with the IFT mutants. Generally, in IFT mutants, cilia are formed with different degrees of abnormality depending on the mutation: shorter, rounder or of normal length but with bulges near the tip [42] . By contrast, the cilia are not formed in the Cc2d2a mutant, suggesting that CC2D2A is required at an early step of ciliogenesis. IFTs are utilized as transport modules at a later stage to build and maintain the cilia. The Shh pathway is initiated in primary cilia for both neural tube and limb bud patterning [22] , [23] . Notably, Shh signalling is perturbed in the developing Cc2d2a −/− neural tube (see Fig. 3b ). Ventral progenitor domains marked by Shh and Olig2 are absent in Cc2d2a −/− embryos. Nkx2.2 is shifted and confined to the floor plate, and both Nkx6.1 and Pax6 show a slight shift towards the ventral midline. These data indicate lost floor plate and diminished V3 progenitor domain, both of which require high levels of Shh signalling for induction. On the other hand, dorsal and lateral fates are largely unaffected in Cc2d2a −/− embryos. The neural tube patterning defect is consistent with reduced Shh signalling and is similar to those reported for Mks1 mutant [25] and some other ciliogenesis or trafficking mutants [23] , [43] . Polydactyly is a common finding in MKS and JBTS [44] , and is caused by aberrant Shh signalling [45] via its effector Gli proteins localized on the ciliary membrane [22] , [46] , [47] . We conclude that both the neural tube defect and polydactyly in Cc2d2a −/− embryos result from a disruption in cilia-based Shh signalling. The two centrioles in the centrosome constitute the primary centre for cytoplasmic MT nucleation, anchoring and elongation in animal cells. Distinct ultrastructural characteristics, specifically the presence of distal appendages and SDA, distinguish the MC from daughter centriole and provide cellular architecture for building the ciliary axoneme using molecular motors and intraflagellar transport [6] , [48] , [49] . Initiation of cilia biogenesis requires the assembly of MT bundles, aster formation and their stabilization at the MC; the absence of CC2D2A will compromise this process. While aberrant immunostaining of ninein, Odf2 and trichoplein indicate a SDA defect, TEM of Cc2d2a −/− MEFs clearly shows the absence or abnormality of SDA. Thus, SDA assembly at the MC requires CC2D2A along with ninein, Odf2 and trichoplein. Odf2 appears to be a core component since SDA are missing in the Odf2 −/− model [28] . Ninein and ε-tubulin are also essential because their depletion halts MT aster formation [50] , [51] . In addition, centriolin and Cep170 are associated with SDA [35] , [52] , although whether they play a direct role is less clear. Additional investigations are required to determine whether distinct proteins are assembled directly at the MC, or if a preassembled complex is attached to the MC to generate SDA. The catalytically inactive transglutaminase-like domain in CC2D2A is a good candidate for providing the MT interaction surface for SDA assembly (see Fig. 8 for a schematic). 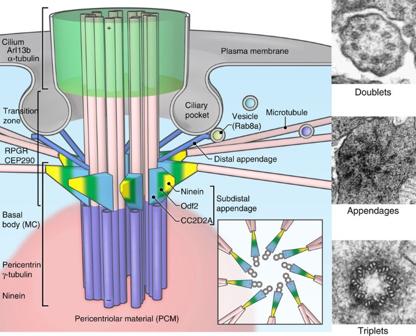Figure 8: A schematic of the base of primary cilium showing the MC (basal body) and the proposed function of CC2D2A at SDA. The MC includes triplet MTs (purple cylinders) that continue as the doublet MTs of the axoneme (pink cylinders). The plus and minus ends of MTs are marked. The proteins localized to the cilium and MC are indicated. Nine extensions of each MT bundle at the border of MC and transition zone represent the SDA (blue–green–yellow pyramids) and distal appendages (blue rods). The proteins localized to SDA are shown in an order from centre to periphery, based on the current experimental evidence. The SDA anchors MT arrays and helps in the docking of transport vesicles at the base of cilium. The distal appendages help in tethering the MC to the plasma membrane, separating the cilium compartment from the cytoplasm. The green circle at the far end of the distal appendage, on the right side, represents a Rab8a-tagged vesicle. Rab8a may help tether plasma membrane to distal appendages with support from Odf2 and CC2D2A. Inset shows the top view of MC at the level of SDA, which are shown anchored to MT. The electron micrographs on the right show a cross-sectional view at the level indicated: doublet axoneme (top), at the level of appendages (middle) and triplet MC (basal body) (bottom). Figure 8: A schematic of the base of primary cilium showing the MC (basal body) and the proposed function of CC2D2A at SDA. The MC includes triplet MTs (purple cylinders) that continue as the doublet MTs of the axoneme (pink cylinders). The plus and minus ends of MTs are marked. The proteins localized to the cilium and MC are indicated. Nine extensions of each MT bundle at the border of MC and transition zone represent the SDA (blue–green–yellow pyramids) and distal appendages (blue rods). The proteins localized to SDA are shown in an order from centre to periphery, based on the current experimental evidence. The SDA anchors MT arrays and helps in the docking of transport vesicles at the base of cilium. The distal appendages help in tethering the MC to the plasma membrane, separating the cilium compartment from the cytoplasm. The green circle at the far end of the distal appendage, on the right side, represents a Rab8a-tagged vesicle. Rab8a may help tether plasma membrane to distal appendages with support from Odf2 and CC2D2A. Inset shows the top view of MC at the level of SDA, which are shown anchored to MT. The electron micrographs on the right show a cross-sectional view at the level indicated: doublet axoneme (top), at the level of appendages (middle) and triplet MC (basal body) (bottom). Full size image A transition zone membrane complex required to build cilia contains CC2D2A, in addition to other MKS–JBTS-associated proteins such as CEP290, Tectonic1 and B9D1 (ref. 21) [21] . It appears that the SDA region is at the base of the ciliary transition zone where triplet MTs of the MC terminate and doublet MTs of the axoneme begin [4] , [53] , [54] . The overlap in RPGR and CC2D2A immunostaining, reported here (see Fig. 7b ), is consistent with this model (see Fig. 8 ) and with their interaction with CEP290 (refs 16 , 55 ); however, these proteins might exist in distinct protein complexes in SDA or transition zone [12] , [14] , [56] . A substantial fraction of mutant MEFs revealed the docking of the MC with the ciliary vesicle but no transition zone was apparent, suggesting a requirement of CC2D2A in transition zone formation ( Fig. 5c , right panel). We hypothesize that CC2D2A interacts with Odf2, which in turn facilitates the delivery of Rab8a vesicles to tether the membrane at the SDA [32] . Accumulation of vesicles observed in Cc2d2a −/− MEFs (see Fig. 5 ) and mislocalization of Rab8 in zebrafish-mutant photoreceptors [31] further support the role of CC2D2A and other SDA proteins in membrane loading and/or tethering during cilia biogenesis. In summary, we demonstrate an essential role of CC2D2A in the formation or stabilization of subdistal appendages to initiate the process of cilia biogenesis from the basal body. Defects in nodal and primary cilia, and consequently Shh signalling, can explain severe pleiotropic phenotypes. Our studies thus provide molecular insights into the MKS disease caused by CC2D2A mutations. Generation of Cc2d2a −/− mice and MEFs for phenotyping All animal experiments were performed after obtaining approval of the animal care and use committee of the National Eye Institute (ASP-NEI 650). The mouse Cc2d2a gene on chromosome 5 spans almost 80 kb and includes 40 exons (gene ID: 231214) with three protein-coding splice variants. Following standard homologous recombination [41] , [57] , exons 6–8 were replaced with a gene-targeting cassette containing homology arms and a β-gal reporter. Southern blotting and PCR validated the correct integration of the targeting cassette. Quantitative reverse transcriptase PCR analysis of different tissues was performed using a TaqMan assay (Applied Biosystems; Mm01211431_m1). The method for RNA-seq analysis of MEFs has been reported [58] . The procedures for electroretinography, histology and immunohistochemistry are reported elsewhere [59] . Analysis of the neural tube for cilia and Shh signalling-associated proteins was largely performed as detailed [43] . MEFs were prepared from E12.5–E13.5 mouse embryos, as instructed (Millipore Tech. Publications). For immunostaining, 70,000 MEFs were plated in each well of a chamber slide (ibidi, WI) with 300 μl of medium. After overnight growth, cilia biogenesis was induced with serum-free medium. The cells were grown to confluence for 48 h, washed with PBS, fixed with 4% paraformaldehyde at room temperature for 15 min and subjected to standard immunostaining protocol. MEFs were imaged on LSM 700 (Zeiss, Germany) confocal microscope, and the images were edited with Adobe Photoshop CS5 and assembled on Adobe Illustrator CS5. The fluorescence intensity in the images was analysed with ImageJ64 (NIH) as performed earlier [60] . Briefly, fluorescence signal (pixel area) in an image was selected with a tool (circle) and integrated density (mean grey value) of the area was measured. Similarly, from the same field, an area with no fluorescence signal (next to a cell) was measured for background intensity. The corrected fluorescence was calculated by the formula, corrected fluorescence=integrated density−(area of pixel with signal × mean fluorescence of background readings). Statistical analysis of difference in fluorescence intensity was performed by t -test (two-tailed, type 2) in Excel (Microsoft). Antibodies The following primary antibodies were used: anti-CC2D2A (Rb,1:300, custom made), anti-acetylated α-tubulin (Ms, 1:500; Sigma, T6793), anti-α-tubulin (Ms, 1:2,000; Sigma, T6199 (DM1A)), anti-γ-tubulin (Ms, 1:500; Sigma, T6557), anti-GT335 (Ms, 1:500; Adipogen, AG-20B-0020), anti-Arl13b (Rb, 1:500; Proteintech, 17711-1-AP;), anti-trichoplein (Rb, 1:100; Masaki Inagaki), anti-human cenexin (ODF2 Rb, 1:50; Kyung Lee), anti-ninein-L77 and –L79 (Rb, 1:2,500; Michel Bornens), anti-Rab8a (Rb, 1:250; Proteintech, 55296-1-AP), anti-rootletin6 ( Rb, 1:500; Tiansen Li) and anti-RPGR-S3 (Chk, 1:300; Tiansen Li), anti-pericentrin (Rb, 1:500; Abcam, ab448), Anti-Olig2 (Rb, 1:200; R&D, AF2418). The following monoclonal antibodies were used (Ms, 1:200, DSHB): Shh, Nkx2.2, Nkx6.1 (clone F55A10), HB9, Msx2, Islet-1 (clone 40.2.D6) Pax6 and Pax7. The secondary antibodies for immune-fluorescence analysis were coupled to Alexa Fluor 488 or 568 dyes (Molecular Probes). MT regrowth assay MEFs were plated at a high confluence onto the chamber slide (70–80%) and the following day, the cells were treated with 5 μM nocodazole (Sigma) in complete media (DMEM) and incubated for 1.5 h at 37 °C. Subsequently, the media was aspirated and the cells were washed once with PBS and replaced with complete media. After treatment, the cells were fixed at time points of interest with 100% methanol 3 min on ice and then processed for immunofluorescence staining, with anti-γ-tubulin and anti-α-tubulin, sequentially. The images were captured on LSM 700 confocal microscope (Zeiss, Germany). Scanning electron microscopy Embryos (E8) were fixed in paraformaldehyde (4%) and glutaraldehyde (2%) in cacodylate buffer (0.1 M) for 2 h at room temperature and then washed in cacodylate buffer thrice (10 min each). The embryos were treated for 1 h in osmium tetroxide (1%), washed thrice (10 min each) in cacodylate buffer and dehydrated in graded ethanol (35%, 50%, 70%, 95%, two times for 10 min each, and then three times with 100%). After treating with tetramethylsilane solution (three times for 10 min each), the embryos were mounted on a SEM stub and sputter coated with gold/palladium using an EMITECH K575 high-resolution coater. Imaging was performed on S-3000N scanning electron microscope (Hitachi, Japan). TEM and immuno-EM The serum-starved MEFs were fixed and processed for TEM as described [61] . Sections of cells in Epoxy blocks (80 nm) were prepared with Leica UCT Ultramicrotome, mounted on 200 mesh copper grids and coated with carbon. The sections were imaged using H-7600 transmission electron microscope (Hitachi). Post-embedding immuno-EM The procedure of post-embedding immuno-EM was previously described [62] . Briefly, cultured IMCD3 cells (CRL-2123, ATCC) were fixed in phosphate-buffered saline containing formaldehyde (4% v/v) and glutaraldehyde (0.05% v/v) for 2 h, then dehydrated in a series of cold ethanol (35%, 50%, 70%, 95% and 100%). The cells were infiltrated in 1:1 and 1:2 mixtures of 100% ethanol and LR White resin for 1 h each, then in LR White resin overnight. The cells were embedded in LR White resin and cured in a 55 °C oven for 24 h. Thin sections (90–100 nm) were then mounted on 300-meshed nickel grids that were first blocked by a commercial blocking buffer for goat antibodies and then incubated in a serial dilution of primary antibody, followed by immunogold-conjugated secondary antibody (10 nm particles). The grids were washed in Tris buffer (pH 7.4) containing BSA (0.1% w/v), NaCl (250 mM) and Tween-20 (0.01% v/v). The grids were stained in uranyl acetate and lead citrate and examined by electron microscope. Post-embedding immunolabelling of monkey photoreceptors Monkey eyes ( Macaca mulatta ) were obtained from the Washington National Primate Research Centre at the University of Washington. Eyes were fixed in 2% paraformaldehyde and 0.5% glutaraldehyde in phosphate buffer for 1 h, then en bloc stained in uranyl acetate, dehydrated and infiltrated in LR White as previously described [63] . Thin sections were collected on nickel grids, blocked in normal goat serum and incubated in anti-CC2D2A antibody (1:100) for 2 h, washed and incubated in goat anti-rabbit 10 nm gold secondary for 1 h. Sections were stained with uranyl acetate and lead citrate and examined on a JEOL 1010 transmission electron microscope. Negative controls (no primary) were run in parallel. Flow cytometry DNA content was assayed by flow cytometry using propidium iodide. Samples were acquired using a FACSCalibur (BD Bioscience, CA) and the data analysed with FlowJo V9.5 (TreeStar, OR) using Watson Pragmatic Modeling. How to cite this article : Veleri, S. et al. Ciliopathy-associated gene Cc2d2a promotes assembly of subdistal appendages on the mother centriole during cilia biogenesis. Nat. Commun. 5:4207 doi: 10.1038/ncomms5207 (2014).